Use of domesticated pigs by Mesolithic hunter-gatherers in northwestern Europe Mesolithic populations throughout Europe used diverse resource exploitation strategies that focused heavily on collecting and hunting wild prey. Between 5500 and 4200 cal BC, agriculturalists migrated into northwestern Europe bringing a suite of Neolithic technologies including domesticated animals. Here we investigate to what extent Mesolithic Ertebølle communities in northern Germany had access to domestic pigs, possibly through contact with neighbouring Neolithic agricultural groups. We employ a multidisciplinary approach, applying sequencing of ancient mitochondrial and nuclear DNA (coat colour-coding gene MC1R ) as well as traditional and geometric morphometric (molar size and shape) analyses in Sus specimens from 17 Neolithic and Ertebølle sites. Our data from 63 ancient pig specimens show that Ertebølle hunter-gatherers acquired domestic pigs of varying size and coat colour that had both Near Eastern and European mitochondrial DNA ancestry. Our results also reveal that domestic pigs were present in the region ~500 years earlier than previously demonstrated. The spread of domesticated plants and animals throughout Europe between 6000 and 4000 cal BC involved a complex social and economic interplay between indigenous Mesolithic hunter-gatherers and incoming Neolithic farmers. Although contacts between these two groups were a feature of the social landscape [1] , [2] , [3] , the conduits through which the exchange and transfer of particular technological, subsistence and social elements might have occurred, and the scale of interaction remain hotly debated. More specifically, evidence regarding the degree to which local hunter-gatherers acquired elements of the introduced Neolithic farming ‘package’, or took ideas from their Neolithic neighbours and independently developed certain aspects of subsistence technologies, are controversial [4] . In northern Europe, a number of claims have been made regarding the possibility that some hunter-gatherers had access to domestic animals [5] , [6] . Of the dozen or so previous assertions made for the presence of domestic sheep, goat, cattle or pig in Mesolithic contexts from Denmark, northern Germany, Poland and the Netherlands, almost all fail scrutiny in terms of their postulated early dates or their identification as domestic animals [5] , [6] ( Supplementary Table S1 ). Interestingly, the only convincing cases to date are both from Ireland, where domestic cattle bones were recovered from late Mesolithic deposits (~4300 cal BC) at Ferriter’s Cove and the slightly younger site at Kilgreany Cave [5] , [7] . Although these remains have been interpreted as the likely importation of joints of meat rather than live cattle [8] , they clearly indicate late Irish Mesolithic links with continental European farmers at a time when no other evidence for such a connection exists in the archaeological record for Britain [9] . There remains as yet, however, no convincing evidence in continental northern Europe that late Mesolithic hunter-gatherers had access to domestic animals other than dogs [5] . In the archaeological record of northern Europe, a long period of coexistence ( circa 5500–4200 cal BC) has been documented between late Mesolithic groups and fully agricultural early Neolithic communities [1] , [2] , [3] . Of particular relevance is the Ertebølle hunter-gatherer culture of southern Scandinavia and northern Germany. In the southern part of their distribution range, the Ertebølle existed in close geographic proximity to Neolithic agricultural communities, first to the Linienbandkeramik (LBK; 5700/5600–4900 cal BC) and later on to the post-LBK communities (Stichbandkeramik 4900–4500 cal BC and Rössen 4500–4200 cal BC) [3] , [10] , [11] , [12] , [13] . Some sporadic communication between these cultures is suggested by the presence in Ertebølle settlements of Danubian type or amphibolite axes and pottery exhibiting decoration styles similar to those frequently portrayed on LBK and Stichbandkeramik ceramics [3] , [10] , [11] , [12] , [13] . However, in this potential ‘zone of interaction’, the Ertebølle appear to have maintained their own hunter-gatherer lifeway, distinct from their agricultural neighbours, likely resisting LBK and post-LBK acculturation altogether [3] , [10] , [11] , [12] , [13] , [14] . Although Ertebølle subsistence was heavily oriented towards the exploitation of marine resources, wild ungulates-especially pigs ( Sus scrofa )-provided an important supplement to the diet [15] , [16] , [17] . Sus bones comprised on average ~30% of Ertebølle game assemblages [15] , [16] , [17] . Traditional biometrical analyses of Ertebølle pig skeletal remains indicated that these animals were mainly large-bodied, and therefore were probably wild boar [4] , [15] , [16] , [17] . Although a single small ‘domestic’ pig has been claimed from the site of Grube–Rosenhof, its ‘domestic’ attribution has been called into question [5] , as the identification is based on a scapula column length measurement, a dimension that in pigs is subject to considerable growth during the life of the animal [18] . As a result, convincing evidence for domestic pigs has yet to be reported from Ertebølle sites before ~4200 cal BC [3] , [4] , [5] , [6] , [15] , [16] , [17] . In contrast, the contemporary Neolithic farming economy was characterized by intensive exploitation of domestic plants and animals such as sheep, goat, cattle and pigs [4] , [19] , [20] , [21] . Although early Neolithic (LBK) domestic sheep and goats clearly originated from the Near East—as no wild progenitors of these species existed in Europe [21] —it is possible that domestic cattle and pigs may have had a local origin because of the Pan-Eurasian distribution of wild aurochsen and boar. Although genetic studies are revealing a detailed picture of cattle [20] , [21] , [22] , [23] and pig [24] , [25] , [26] exploitation by early Neolithic farmers, none have been directed towards exploring whether the Mesolithic Ertebølle hunter-gatherers of northern Germany acquired domestic animals (directly or indirectly) from their early or middle Neolithic neighbours to the south. To address this question, we applied ancient DNA (aDNA) analysis to Sus remains recovered from Ertebølle, LBK and post-LBK settlements in temporal association, including the site of Rosenhof where previous disputed claims for the presence of both domestic cattle and pigs have been made [3] , [5] , [6] . An 80-bp fragment of the maternally inherited mitochondrial control region (from which phylogeographic information about the origin of the sampled animals can be inferred [26] , [27] , [28] ) was successfully analysed in 63 out of 144 bone and tooth samples. The haplotype information derived from this fragment permits separation of pigs of Near Eastern-and (in this case) certainly domesticated-ancestry from those of European origin. In addition, variation in the MC1R gene, associated with different coat colour patterns, was successfully sequenced for seven specimens. Spotted coat colour phenotypes are commonly seen in many modern domestic breeds [29] , [30] , [31] , [32] , [33] . A recent study determined that all known MC1R mutations in Eurasian wild boar are synonymous, suggesting that MC1R alleles leading to anything other than wild-type camouflage coat colour are quickly eliminated in the wild [32] . As a result, the MC1R gene has been used as a marker of hybridization between wild and domestic Sus [33] and can be used as evidence for domestication in archaeological specimens. Furthermore, geometric morphometric (GMM) analyses were carried out on all corresponding specimens where molar teeth were present ( N =92), to use molar shape to assess their wild or domestic status [34] and contrast the results with traditional biometrics [35] and aDNA results. The combination of a genetic and morphometric approach applied to the 63 pig remains shows that Ertebølle hunter-gatherers acquired domestic pigs of varying size and coat colour that had both Near Eastern and European mitochondrial DNA (mtDNA) ancestry. Our results reveal that the northern European Mesolithic Ertebølle hunter-gatherers did not only possess domestic pigs like those of their agricultural neighbours, but that these animals were present in the region ~500 years earlier than has been previously demonstrated. The mtDNA sequences from the specimens recovered from LBK and post-LBK ( N =37) and Ertebølle ( N =26) sites in Germany ( Fig. 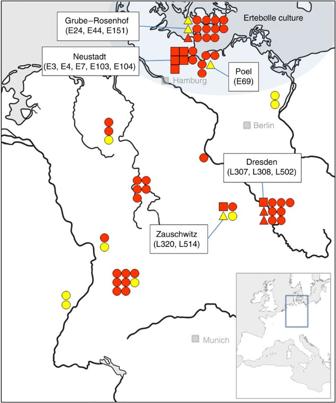Figure 1: Map depicting the location of the archaeologicalSussamples from which mtDNA haplotypes were obtained. Samples were recovered from Neolithic LBK, post-LBK and Mesolithic Ertebølle sites dated between 5500 and 4000 cal BC. Each symbol corresponds to a single sample (triangle, square and circle). Domestic (triangle) and wild (square) pigs discussed in the text are labelled; circles representSusspecimens of unknown domestication status. The red colour indicates the European haplotypes C and A, and yellow the Near Eastern haplotypes Y1 and Y2. 1 , Table 1 ) clustered into four previously described clades ( Fig. 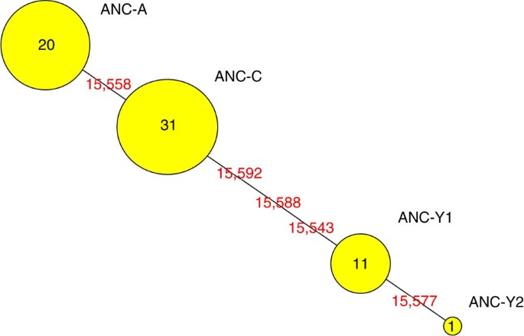Figure 2: The phylogenetic network based on haplogroups determined by the 80-bp-long diagnostic control region fragment of mtDNA. The phylogenetic network was constructed using the program Network45. The size of the circles is proportional to the number of individuals in each haplogroup—numbers are shown in the circles. Distances between the circles correspond to the number of mutations (positions indicated by red numbers) between the haplotypes. 2 , Table 2 , Supplementary Data 1 ) [24] , [26] : the Near Eastern haplotypes Y1 (17.5%, N =11) and Y2 (1.6%, N =1) and the European branches A (31.7%, N =20) and C (49.2%, N =31; Table 1 , Supplementary Data 2 ). LBK, post-LBK and Ertebølle sites share similar compositions of Near Eastern and European Sus haplotypes (Fisher’s test, P =0.3; Table 1 , Supplementary Data 2 ) but Ertebølle Sus have significantly larger molars (the Kruskal–Wallis test, P <0.05; Fig. 3 ). Figure 1: Map depicting the location of the archaeological Sus samples from which mtDNA haplotypes were obtained. Samples were recovered from Neolithic LBK, post-LBK and Mesolithic Ertebølle sites dated between 5500 and 4000 cal BC. Each symbol corresponds to a single sample (triangle, square and circle). Domestic (triangle) and wild (square) pigs discussed in the text are labelled; circles represent Sus specimens of unknown domestication status. The red colour indicates the European haplotypes C and A, and yellow the Near Eastern haplotypes Y1 and Y2. Full size image Table 1 Summary of mtDNA results of archaeological Sus samples. Full size table Figure 2: The phylogenetic network based on haplogroups determined by the 80-bp-long diagnostic control region fragment of mtDNA. The phylogenetic network was constructed using the program Network [45] . The size of the circles is proportional to the number of individuals in each haplogroup—numbers are shown in the circles. Distances between the circles correspond to the number of mutations (positions indicated by red numbers) between the haplotypes. Full size image Table 2 Variations of the 80-bp control region fragment of mtDNA used for phylogeographic analyses. 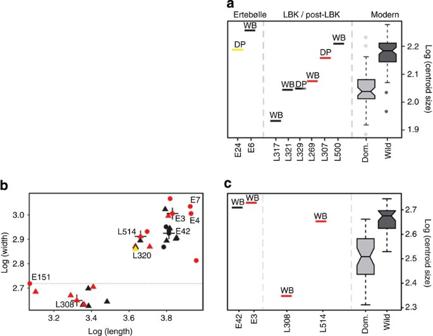Figure 3: Size variation of archaeological compared with modernSusspecimens. AncientSussamples compared with modern wild and domestic (Dom.) pigs for the lower second (a) and third (b,c) molars calculated using traditional metrics (b) and GMMs (a,c). Specimens analysed by both techniques are identified by a cross inb. Where it was possible to identify specimens by their molar shape, they have been labelled as either domestic pig (DP) or wild boar (WB). Red indicates the European haplotypes C and A, yellow the Near Eastern haplotypes Y1 and Y2. Black represents specimens for which no aDNA results were obtained. Full size table Figure 3: Size variation of archaeological compared with modern Sus specimens. Ancient Sus samples compared with modern wild and domestic (Dom.) pigs for the lower second ( a ) and third ( b , c ) molars calculated using traditional metrics ( b ) and GMMs ( a , c ). Specimens analysed by both techniques are identified by a cross in b . Where it was possible to identify specimens by their molar shape, they have been labelled as either domestic pig (DP) or wild boar (WB). Red indicates the European haplotypes C and A, yellow the Near Eastern haplotypes Y1 and Y2. Black represents specimens for which no aDNA results were obtained. Full size image The presence of Near Eastern Sus haplotypes in the LBK confirms previous observations that domesticated pigs of Near Eastern ancestry were introduced to Europe during the Neolithic period [24] , [25] . More surprising is the presence of three Ertebølle pigs from Grube–Rosenhof (specimens: E24, E44) and Poel (E69) from northern and northeastern Germany that possessed the Near Eastern haplotype Y1 ( Table 3 , Supplementary Data 1, 2 ). This result indicates the presence of animals with an ‘exotic’ domestic origin in a hunter-gatherer context ( Fig. 1 , Table 3 ). In addition, one of these specimens (E24) revealed a range of other domestic traits: (a) homozygous for the MC1R E p allele 501, showing that the animal possessed a ‘black spotted’ coat colour, a domestic phenotype ( Table 3 , Supplementary Data 3 ); (b) GMM analyses of the second lower molar revealed a ‘domestic shape’ classification; and (c) the lower third premolar was rotated ( Fig. 4 ), a pathology observed more often in domestic than in wild animals [16] , [17] . Finally, direct dating of E24 (4720–4582 cal BC, KIA 41338) confirmed its younger Ertebølle cultural affiliation (~4750–4450 cal BC) [3] . Table 3 Identification of wild boar and domestic pigs in Ertebølle and agricultural sites. 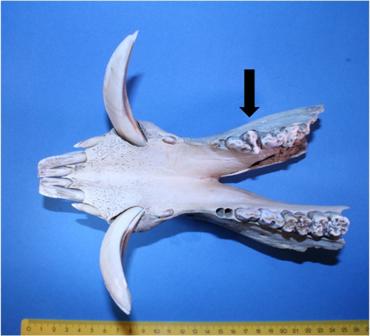Figure 4: Occlusal view of mandible. Specimen number E24. The rotated lower third premolar is indicated by an arrow. Measurement scale is in centimetres. Full size table Figure 4: Occlusal view of mandible. Specimen number E24. The rotated lower third premolar is indicated by an arrow. Measurement scale is in centimetres. Full size image Although genetics, phenotype and pathology all strongly indicate that E24 represents the remains of a domestic animal, traditional biometry shows the specimen was very large ( Fig. 3 ), falling within the modern-day size distribution of German wild boar and markedly outside that of modern European domestic pigs. A similarly large specimen (L320)—carrying the Near Eastern Y1 haplotype ( Fig. 3 , Table 3 ) and classified by GMM analyses as a ‘domestic’ pig shape—was identified at the Neolithic site of Zauschwitz in eastern Germany, further underscoring the unreliability of molar size as a definitive marker for domestic or wild status [34] . As Ertebølle and Neolithic groups (LBK, Stichbandkeramik and Rössen) coexisted for ~700 years (between 5500 and 4200 cal BC) [1] , [2] , [3] , [12] , [13] , the presence of a domestic pig dated from 4720 to 4582 cal BC at an Ertebølle site suggests that contact was frequent enough to be detected in the limited sample size analysed in this study. It seems that specimen E24 represents the earliest evidence of the first domesticated pigs introduced to the region. By far the most frequent Sus mtDNA haplotypes in both LBK and post-LBK ( N =28) and Ertebølle ( N =23) sites are European haplogroups A and C [26] , [28] . As previous genetic evidence suggests that European wild boar were incorporated into domestic stocks soon after the introduction of Near Eastern pigs, individuals carrying European haplotypes could be either wild or domestic animals. As a result, mtDNA sequences alone cannot be used to determine domestic or wild status in European suids. Using a combined genetic and morphometric approach, however, it was possible to more confidently assign status calls. For example, the combination of a European mtDNA haplotype, an MC1R allele associated with wild coat colour and/or a wild tooth shape was interpreted as wild boar. Five Ertebølle (E3, E4, E7, E103 and E104) and two LBK/post-LBK (L502 and L514) specimens possessed this combination of criteria ( Fig. 3 , Table 3 ). Although size can be a misleading indicator of domestication status [36] , the presence of pigs smaller than modern wild boar that possessed European haplotypes found in both LBK and Ertebølle sites ( Fig. 3 , Table 3 ) was unexpected. One of these specimens (E151) from the Ertebølle site of Grube–Rosenhof in northern Germany also carried the MC1R mutation associated with domestic coat colour. A small LBK specimen with a European mtDNA lineage (L308) from Dresden, Brodau in eastern Germany possessed a tooth shape more similar to wild boar than domestic pig. Another European LBK specimen (L307) from the same site represented a larger individual and possessed a domestic tooth shape. The wide disparities in molar size and shape present in these animals suggest that these traits provide a different signal of domestication for these European S. scrofa remains ( Table 3 ). A previous study concluded that European mtDNA haplotypes appeared in domestic swineherds around 4000 cal BC, and then rapidly proliferated to become the dominant haplotype [26] , [27] . Although not directly dated, specimen E151—an animal of European mtDNA lineage exhibiting a domestic coat colour—derives from a context dated by 14 C to between 4900 and 4400 cal BC [3] , making it the earliest domesticated pig of European wild boar ancestry yet identified. These data suggest that the process of local domestication of European wild boar is perhaps 500 years earlier than previously recognized and was at least initiated by central European post-LBK cultures [26] . The fact that this first European domestic pig is in a Mesolithic context reveals evidence that Ertebølle hunter-gatherers had access to and acquired several kinds of domestic pig either directly or indirectly from their post-LBK neighbours (Stichbandkeramik and Rössen). Our results reveal a mixed and complex pattern of pig domestication, livestock management, breeding and cultural interaction between LBK and post-LBK farmers and hunter-gatherer communities in northern Europe. More or less contemporaneously, small and large (or relatively large compared with modern wild boar) domestic pigs of Near Eastern and European origin appeared in Ertebølle, LBK and post-LBK cultural contexts. Whether these pigs correspond to fully domesticated pigs, crosses between wild and domestic pigs, feral animals or pigs at the beginning of the domestication process remains unclear. A loose or more ‘hands-off’ management strategy that encouraged domesticated pigs to forage unsupervised—a practice commonly used in non-intensive husbandry regimes today and in the past [37] —would have resulted in the escape of domestic pigs into the wild where they could have bred with wild boar. Near Eastern mtDNA haplotypes have so far not been observed in ancient or modern European wild boar [26] , [27] , [28] , [30] , [31] , [32] , [33] , [38] , [39] , suggesting that even if this did occur, the wild–domestic crosses have not left a significant mtDNA footprint in ancient or extant indigenous European wild boar populations. The combination of a genetic and morphometric approach applied to the pig remains studied here demonstrates that the northern European Mesolithic Ertebølle hunter-gatherers possessed domestic pigs also kept by their agricultural (Stichbandkeramik and Rössen) neighbours. Whether these hunter-gatherer groups acquired domestic pigs via trade or exchange, or indirectly by hunting or capturing escaped animals remains unknown. What is clear, however, is that the acquisition of domestic pigs by these last hunter-gatherers was one (perhaps critical) component of a broader socioeconomic process by which the Ertebølle acquired and assimilated agricultural elements, eventually leading to the emergence of the Trichterbecher culture. Although it is unclear why the Ertebølle sought domestic pigs, both large and small pigs with multi-coloured coats would likely have seemed strange and exotic compared with the more familiar appearance of the locally available wild boar they traditionally hunted. Whether mere subsistence or other factors led to the acquisition of domestic pigs, it did not immediately revolutionize hunter-gatherer animal exploitation strategies—the Ertebølle still hunted and gathered wild prey for hundreds of years while simultaneously exploiting a few domestic pigs. It did, however, ultimately open a gateway to lifeways centred on the continuous use of livestock as a dietary staple. Whether these two types of domestic pigs derive from the same mixed swineherd remains unknown; however, the genetic and morphometric data strongly suggest that early agriculturists employed a complex management and breeding strategy for suids. Rather than a simple developmental trajectory of exploitation from wild to domestic animals, our data suggest that both the domestication process and associated management scenarios were much more complex and involved than previously imagined. What is clear is that these domestic pigs do, however, represent not only the first domestic animals identified from Mesolithic sites in continental northern Europe, but also the earliest domesticates from the region—appearing some 500 years before the first reliable evidence for domestic cattle, sheep or goat [3] , [4] , [5] , [6] , [16] , [20] , [24] , [25] . aDNA quality control procedures Preparation (that is, cutting, surface decontamination and grinding) of bones and teeth, DNA extraction and pre-PCR processing were performed in three separate rooms dedicated to aDNA procedures, following established stringent protocols [40] , [41] , [42] . No modern DNA-based studies had ever been performed before in the rooms. All procedures were carried out in ultraviolet-irradiated DNA workstations. Access to the laboratory and handling of the archaeozoological material were limited to authorized personnel only. Post-PCR work was routinely conducted in facilities different from those where aDNA was processed. Contamination prevention steps included the use of ultraviolet-irradiation, PCR workstations, disposable coveralls, masks and gloves [40] , [41] , [42] . Workbenches and surfaces were always bleached before experimental procedures. Only sterile RNA/DNA-free manufactured plasticware and filter tips in small packaging units were used. Disposable consumables and most of the solutions, buffers and ddH 2 O were irradiated with ultraviolet-light covered with aluminium foil [43] . Negative controls were employed in all experimental steps (grinding, DNA extraction, pre-PCR preparation, PCR and sequencing) to rule out recent contamination. Primers applied in this study were specific for the genus Sus and showed no amplification success with DNA from humans or other animal species such as cattle, horse, cat or dog. A subset of four bone and tooth specimens was sent to the Ancient DNA Laboratory in Durham (UK), where for each case the mtDNA findings were verified ( Supplementary Data 1,2 ). Sample preparation and DNA extraction Bones and teeth of 144 Sus specimens were investigated from 17 archaeological sites in Germany ( Supplementary Data 1, 2 ). The surface of all samples was sanded down with a circular saw and bleached to remove external contaminants. Samples were ground to fine-grained powder. DNA was extracted by a magnetic bead-based technology using the Biorobot-EZ1 (Qiagen, Hilden, Germany) [44] . For each individual, a minimum of two independent DNA extractions were performed. mtDNA sequence analysis An 80-bp-long diagnostic fragment from the control region of the Sus mitochondrial genome was amplified using two primer combinations ( Supplementary Table S2 ). Amplicons ranged from 128 to 173 bp in size and contained polymorphic sites that were used to define haplogroups and haplotypes. The amplification was carried out as singleplex PCR in a final volume of 25 μl ( Supplementary Table S3 ). The amplification was performed in a Mastercycler (Eppendorf, Hamburg, Germany) under the following conditions: initialization at 94 °C for 11 min; 35–42 cycles at 94 °C for 30 s, 52 °C for 30 s, 72 °C for 30 s and a final elongation step at 72 °C for 10 min. The amplification success was controlled by electrophoresis on a 2% agarose gel. Subsequently, 5 μl of the PCR products were treated with 2 μl ExoSAP-IT (USB, Affymetrix, Freiburg, Germany) in a Mastercycler at 37 °C for 15 min and at 80 °C for 15 min. The products were subjected to direct sequencing using the BigDye Terminator v3.1 Kit (Applied Biosystems, Foster City, USA). The sequencing conditions followed the instructions of the manufacturer. Sequencing products were purified applying the DyeEx 2.0 Spin Kit (Qiagen) and analysed using the ABI Prism 310 and 3130 Genetic Analyzers (Applied Biosystems). Sequences were aligned and verified manually with the programs DNA-Alignment [45] , DNAStar (Lasergen 8.0) and Bioedit (7.0.9). From each bone/tooth sample, a minimum of two extracts were prepared. For each extract that yielded amplifiable DNA, sequences were obtained independently at least twice. Only those samples that showed amplicons in more than one extract were considered for further analyses. Coat colour analysis Six fragments of the MC1R gene were amplified to determine 14 nucleotide variations known to be associated with changes in coat colour in modern European pig breeds [31] ( Supplementary Table S4 ). The PCR primer sets are listed in Supplementary Table S5 . The amplifications were carried out in singleplex PCRs in a final volume of 25 μl ( Supplementary Table S6 ). 7-deaza-2′-deoxyguanosine was used in the amplification to improve the processing of GC-rich regions [46] . The amplification was performed in a Mastercycler (Eppendorf) under the following conditions: initialization at 94 °C for 11 min; 15 cycles at 94 °C for 30 s, 60 °C for 30 s+1 °C per cycle, 72 °C for 30 s; 25–27 cycles at 94 °C for 30 s, 60 °C for 30 s, 72 °C for 30 s and a final elongation step at 72 °C for 10 min. The amplification success was tested using gel electrophoresis followed by direct sequencing (see above). To confirm the results, the 14 MC1R variants were also typed employing the single base extension (SBE) method using the SNaPshot Multiplex Kit (Applied Biosystems) [47] . A multiplex PCR in a final volume of 25 μl was performed under the same conditions as for the singleplex approach ( Supplementary Table S6 ). The SBE reactions were carried out using the ABI Prism SNaPshot Multiplex reaction kit (Applied Biosystems) following the manufacturer’s instructions. Two multiplex reactions were designed containing eight and six SBE primers, respectively ( Supplementary Table S7 ), to increase the efficiency and sensitivity of the protocol for the analysis of highly degraded DNA. The components of the reaction mixes are reported in Supplementary Table S8 . The cycling conditions are an initial step at 96 °C for 6 min, followed by 25 cycles of denaturation at 96 °C for 10 s, annealing at 55 °C for 5 s and elongation at 60 °C for 30 s. Sequencing products were run on ABI Prism 310 and 3130 Genetic Analyzers (Applied Biosystems). The resultant electropherograms were analysed using GeneMapper version 3.2 Software (Applied Biosystems). Subsequently, the allelic status of the 14 loci was determined to infer the individual coat colour [31] . Verification of mtDNA results in Durham DNA extraction was performed in the Ancient DNA Laboratory in the Archaeology Department at Durham University following strict laboratory procedures according to commonly applied guidelines [40] , [41] , [42] . All equipment and work surfaces were cleaned before and after each use with a dilute solution of bleach (10%) followed by ethanol (99%). A strict one-way system for entering the labs is in use to avoid introducing post-PCR contaminants. The ancient pig remains were prepared for DNA extraction by removing a layer of the outer bone surface using a dremel drill with clean cut-off wheels (Dremel no. 409), targeting compact cortical bone. The bone was then pulverized in a micro-dismembrator (Sartorious-Stedim Biotech S.A., Aubagne Cedex, France). Bone powder was digested in 0.425 M EDTA, 0.05% SDS, 0.05 M Tris-HCI and 0.333 mg ml −1 proteinase K, and was incubated overnight on a rotator at 50 °C until fully dissolved. The reagent master mix, excluding proteinase K, was ultraviolet-irradiated at 254 nm for an hour using a crosslinker before suspension in extraction buffer. Two millilitres of supernatant was concentrated in a Millipore Amicon Ultra-4 30 KDa molecular weight cut-off to a final volume of 100 μl. The concentrated extract was purified using the QIAquick PCR Purification Kit (Qiagen) following the manufacturer’s recommendations, with a final elution volume of 100 μl. One negative extraction control was performed alongside five to ten ancient bone samples. PCRs for the mtDNA control region fragments were set up in 25-μl reactions ( Supplementary Table S9 ). One PCR-negative control was included for every 5–8 aDNA template PCRs. PCR cycling conditions were 95 °C for 5 min, 50 cycles of 94 °C for 45 s, 54 °C for 45 s and 72 °C for 45 s, followed by 72 °C for 10 min. Sanger sequencing was performed on the Applied Biosystems 3730 DNA Analyser at the DNA Sequencing Service in the School of Biological and Biomedical Sciences at Durham University. Trace files were manually inspected with 4Peaks (Mekentosj) or Geneious [48] using the assembly function (default parameters). GMM analyses Maximum tooth length and width of molars were measured using a caliper [18] , [35] . Differences in traditional molar size between pig specimens from Ertebølle and LBK sites were tested using Kruskal–Wallis tests. GMM techniques were used to analyse centroid size and shape of lower and upper second and third molars following a standardized protocol [34] , [49] . GMM data correspond to two-dimensional landmark and sliding semi-landmark coordinates that were recorded and analysed [34] . GMM techniques were applied to available archaeological specimens that were identified as ‘wild’ or ‘domestic’ using predictive linear discriminant analyses. The modern reference specimens include 400 teeth corresponding to 73 modern German wild boar and 53 pigs from various European breeds [34] ( Supplementary Table S10 ). Archaeological specimens were labelled as ‘middle’ when showing a centroid size in the overlap of modern wild and domestic pig size, ‘large’ when above, and ‘small’ when below. Coordinates of landmarks and sliding semi-landmarks were acquired with TpsDig2 v2.16 (ref. 50 ). TPS Relw v1.49 (ref. 51 ) was used to slide the semi-landmarks with the Procustes distance minimization criteria, and to superimpose all the specimens using a Generalized Procustes Analysis [52] , [53] . Predictive discriminant analyses were carried out using ‘R’ and ‘Rmorph’ [54] , [55] to allocate the archaeological specimen to one of the two modern reference groups. Traditional size was visualized using biplots and centroid sizes using boxplots. Accession codes : The obtained mitochondrial and nuclear sequences have been deposited in the NCBI GenBank nucleotide database under accession numbers KF274958 – KF275020 and KF418278 – KF418312 . How to cite this article: Krause-Kyora, B. et al. Use of domesticated pigs by Mesolithic hunter-gatherers in northwestern Europe. Nat. Commun. 4:2348 doi: 10.1038/ncomms3348 (2013).